Ultrathin platinum nanowires grown on single-layered nickel hydroxide with high hydrogen evolution activity Design and synthesis of effective electrocatalysts for hydrogen evolution reaction in alkaline environments is critical to reduce energy losses in alkaline water electrolysis. Here we report a hybrid nanomaterial comprising of one-dimensional ultrathin platinum nanowires grown on two-dimensional single-layered nickel hydroxide. Judicious surface chemistry to generate the fully exfoliated nickel hydroxide single layers is explored to be the key for controllable growth of ultrathin platinum nanowires with diameters of about 1.8 nm. Impressively, this hybrid nanomaterial exhibits superior electrocatalytic activity for hydrogen evolution reaction in alkaline solution, which outperforms currently reported catalysts, and the obviously improved catalytic stability. We believe that this work may lead towards the development of single-layered metal hydroxide-based hybrid materials for applications in catalysis and energy conversion. Outstanding energy storage density and perfect environmental friendliness make hydrogen an ideal energy carrier or clean fuel [1] , [2] . Among different strategies to produce hydrogen, alkaline water electrolysis has been receiving special attention due to its unique advantages including unlimited reactant availability, good manufacturing safety, stable output and high product purity [3] , [4] , [5] , [6] , [7] . However, the sluggish kinetics of hydrogen evolution reaction (HER) in a basic environment (2H 2 O+2e→H 2 +2OH − ) causes high overpotential and associated large energy consumption, which greatly hinder practical application of alkaline electrolysis [8] . As a typical example, though platinum (Pt) is generally believed as one of the best electrocatalysts for HER, its catalytic activity is about two orders of magnitude lower in alkaline environment compared with that in acidic electrolyte [8] , [9] , [10] , [11] , [12] , [13] , [14] , [15] , [16] , [17] , [18] . A plausible way to enhance the HER activity of Pt in basic media is a combination of Pt with metal hydroxides, that is, electrochemical deposition of ultrathin Ni(OH) 2 nanoclusters on Pt electrode surfaces [8] , [19] , [20] , [21] , [22] , [23] . In this type of hybrid materials, the edges of the Ni(OH) 2 clusters promote dissociation of water and production of hydrogen intermediates, which subsequently adsorb on the nearby Pt surfaces and recombine into molecular hydrogen [8] . These pioneering works hold the promise that the sluggish kinetics of HER might be circumvented if rational fabrication of the hybrid materials could be accomplished and the synergetic interactions between noble metal and metal hydroxide are exploited. However, unlike many reports on successful deposition of noble metal nanoparticles (NPs) on 2D graphene oxide (GO) sheets [24] , [25] , [26] , [27] , controllable growth of noble metal NPs on the layered metal hydroxide sheets is rarely realized. The difficulty lies in the fact that, with respect to the GO sheets, much fewer surface functional groups (like carboxylic acid and carbonyl) result in the reduced adsorption of noble metal ions onto the metal hydroxide sheets, making it unfavourable for heterogeneous nucleation and growth of noble metal NPs on the surface of the layered metal hydroxides. In this work, we report a design strategy in which we grow one-dimensional (1D) ultrathin Pt nanowires (NWs) on two-dimensional (2D) Ni(OH) 2 nanosheets to construct the high performance catalysts for HER in basic solution. We demonstrate that single-layered Ni(OH) 2 (SL-Ni(OH) 2 ) nanosheets with the suitable surface modification are the key to immobilization and growth of ultrathin Pt NWs (defined as Pt NWs/SL-Ni(OH) 2 ), and the obtained Pt NWs/SL-Ni(OH) 2 hybrid materials exhibit unprecedented catalytic activity and stability towards HER in basic solution. Unlike previous reports involving utilization of Pt electrodes [8] , [19] , [20] , [21] , [22] , the selection of single-layered 2D Ni(OH) 2 (SL-Ni(OH) 2 ) nanosheets as the substrates is based on cost considerations [28] , [29] , as SL-Ni(OH) 2 sheets might be cheaply acquired via exfoliation of lamellar α-Ni(OH) 2 (refs 30 , 31 , 32 , 33 ). Furthermore, compared with commonly used zero-dimensional (0D) Pt nanoparticles (NPs), 1D ultrathin Pt NWs of high aspect ratios, few lattice boundaries and smooth crystal planes offer the opportunity for improvement of the catalytic activity [34] , [35] , [36] , [37] , [38] , [39] , [40] , [41] , [42] , [43] , [44] . Meanwhile, a large contact area between Pt NWs and the Ni(OH) 2 substrates can effectively alleviate possible migration and aggregation of Pt NWs and thus benefit enhancement of the catalytic stability [40] . Growth of ultrathin Pt nanowires on single-layered Ni(OH) 2 The synthesis procedure of Pt NWs/SL-Ni(OH) 2 is schematically depicted in Fig. 1a . First, well-dispersed SL-Ni(OH) 2 nanosheets in formamide were prepared by exfoliation of layered Ni(OH) 2 intercalated with dodecyl sulfate (DS) ions [33] . The single-layered nature of the exfoliated SL-Ni(OH) 2 nanosheets was confirmed by the corresponding atomic force microscopy (AFM) measurement ( Supplementary Fig. 1 ). Subsequently, 300 μl K 2 PtCl 4 (60 mM) and 50 μl KOH (5 M) aqueous solutions were added to 10 ml SL-Ni(OH) 2 formamide dispersion (0.5 mg ml −1 ), respectively. Finally, the mixture was subjected to solvothermal treatment in a 20-ml Teflon-lined autoclave at 120 °C for 4 h to obtain the Pt NWs/SL-Ni(OH) 2 hybrids. In this synthesis, formamide acts as both the solvent for dispersing SL-Ni(OH) 2 nanosheets and the reducing agent for generation of Pt NWs [33] , [45] . 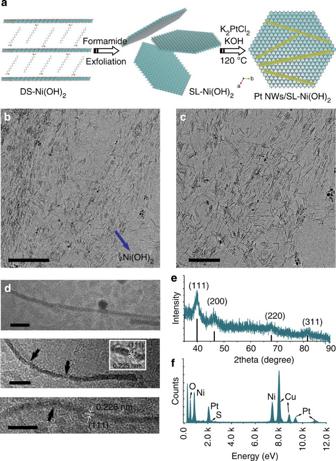Figure 1: Schematic illustration of synthesis procedure and the resulting Pt NWs/SL-Ni(OH)2. (a) Scheme for synthesis of Pt NWs/SL-Ni(OH)2; (b–d) TEM images of Pt NWs/SL-Ni(OH)2, scale bars in (b), (c) and (d) are 100, 50 and 5 nm, respectively; (e) XRD pattern of Pt NWs/SL-Ni(OH)2along with the corresponding JCPDS standard of Pt; (f) EDX spectrum of Pt NWs/SL-Ni(OH)2. Note that the Cu signal in (f) originates from the TEM grid used. Figure 1b,c presents the typical transmission electron microscopy (TEM) images of as-synthesized products. It is evident that the Pt nanostructures are exclusively formed on the surface of SL-Ni(OH) 2 nanosheets, and about 94% Pt nanostructures are 1D ultrathin NWs with the uniform diameters of ~1.8 nm and varying lengths of 10 to 50 nm ( Supplementary Fig. 2 ). We also note that both the SL-Ni(OH) 2 substrates and the immobilized ultrathin Pt NWs are very sensitive to the electron beam during TEM analysis, and many breakages are discerned when exposed to the electron beam ( Supplementary Fig. 3 ). High-resolution TEM image indicates that the ultrathin Pt NWs are composed of multiple crystalline segments with the lengths of 5 to 10 nm (black arrows in Fig. 1d ). The crystallinity characteristics of Pt NWs are further investigated by X-ray diffraction (XRD) pattern, in which the diffraction peaks can be indexed to (111), (200), (220) and (311) reflections of face centred cubic ( fcc ) Pt (JCPDS No. 87-0647), respectively ( Fig. 1e ). The XRD result also excludes formation of Pt-Ni alloy [46] . The Ni(OH) 2 -Pt contact area in Pt NWs/SL-Ni(OH) 2 is qualitatively measured by determining the electrochemical surface area (ECSA) of Pt NWs within Pt NWs/SL-Ni(OH) 2 and Pt NWs completely exposed after removing SL-Ni(OH) 2 ( Supplementary Figs 4–6 and Supplementary Note 1 ). The contacted part of Pt NWs with SL-Ni(OH) 2 deduced from their ECSA result is ~35%, and hence the exposed Pt atoms account for ~65%. Figure 1: Schematic illustration of synthesis procedure and the resulting Pt NWs/SL-Ni(OH) 2. ( a ) Scheme for synthesis of Pt NWs/SL-Ni(OH) 2 ; ( b – d ) TEM images of Pt NWs/SL-Ni(OH) 2 , scale bars in ( b ), ( c ) and ( d ) are 100, 50 and 5 nm, respectively; ( e ) XRD pattern of Pt NWs/SL-Ni(OH) 2 along with the corresponding JCPDS standard of Pt; ( f ) EDX spectrum of Pt NWs/SL-Ni(OH) 2 . Note that the Cu signal in ( f ) originates from the TEM grid used. Full size image In addition to the shape and structure, the composition and chemical state of Pt NWs/SL-Ni(OH) 2 are recognized by energy-dispersive X-ray (EDX) spectrum ( Fig. 1f ) and X-ray photoelectron spectroscopy (XPS) ( Fig. 2 ). The EDX analysis clearly distinguishes Pt element from Pt NWs, as well as O and Ni elements from SL-Ni(OH) 2 nanosheets ( Fig. 1f ). Interestingly, small amount of S element is also detected in EDX spectrum, revealing the adsorption of DS ions on the surface of SL-Ni(OH) 2 sheets. Deconvolution of Pt 4f XPS doublet (4f 7/2 and 4f 5/2 ) gives rise to two pairs of peaks, corresponding to dominant Pt (0) atoms (82.9%, green curves in Fig. 2a ) and less amount of surface Pt (II) ions (18.1%, red curves in Fig. 2a ), respectively. Another feature coexisted in Pt 4f region is the presence of Ni 3p peaks that are ascribed to Ni (II) species in SL-Ni(OH) 2 (blue curves in Fig. 2a ) [47] , [48] , [49] . It is also discerned by Ni 2p XPS spectra that there is no significant change in the chemical state of Ni (II) after growing Pt NWs on SL-Ni(OH) 2 surfaces ( Fig. 2b ). This phenomenon is coincident with both TEM and XRD observations ( Fig. 1b,c,e ), disclosing that Ni(OH) 2 nanosheets maintain the lamellar structure and do not react with Pt ions to form the alloy after the solvothermal reaction. The total Pt content in Pt NWs/SL-Ni(OH) 2 is about 38.0 wt.%, which is quantitatively measured with a inductively coupled plasma mass spectrometry (ICP-MS) technique. 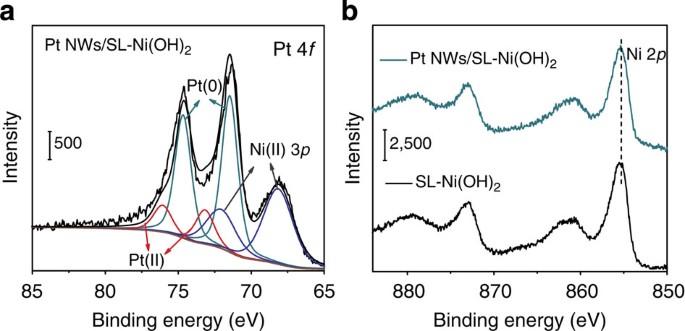Figure 2: XPS analysis of Pt NWs/SL-Ni(OH)2. (a) XPS spectrum of Pt 4f region of Pt NWs/SL-Ni(OH)2; (b) XPS spectra of Ni 2p region of Pt NWs/SL-Ni(OH)2and SL-Ni(OH)2. The dashed line in (b) highlights that the Ni 2p peak position in the two samples remains the same. Figure 2: XPS analysis of Pt NWs/SL-Ni(OH) 2. ( a ) XPS spectrum of Pt 4f region of Pt NWs/SL-Ni(OH) 2 ; ( b ) XPS spectra of Ni 2p region of Pt NWs/SL-Ni(OH) 2 and SL-Ni(OH) 2 . The dashed line in ( b ) highlights that the Ni 2p peak position in the two samples remains the same. Full size image The experimental parameters including the added amount of KOH, reaction temperature and reaction time were investigated in detail for better understanding of formation mechanism of Pt NWs/SL-Ni(OH) 2 hybrid materials. It is found that the reduction rate of Pt precursors by formamide is decreased as the amount of KOH is increased. In the absence of KOH, large amount of Pt NPs is rapidly formed outside the SL-Ni(OH) 2 nanosheets ( Supplementary Fig. 7 ); small amount of adding KOH (5 μl of 5 M KOH solution into 10 ml of 0.5 mg ml −1 SL-Ni(OH) 2 formamide dispersion) gives rise to production of spherical Pt NPs with average diameter of ~3.2 nm on surface of SL-Ni(OH) 2 (Pt NPs/SL-Ni(OH) 2 ) ( Supplementary Fig. 8 ), whereas the reduction of Pt precursors by formamide is hardly happened even after 12 h in the presence of excessive amount of KOH (that is, 100 μl of 5 M KOH solution was added in 10 ml of 0.5 mg ml −1 SL-Ni(OH) 2 formamide dispersion). As shown in Supplementary Fig. 9 , the reaction temperature and duration also have large impact on the final products. The aggregates of ultrathin Pt NWs are formed when the reaction time is prolonged from 4 to 12 h at 120 °C, while Pt NPs assemblies are produced when the reaction temperature is increased from 120 to 140 °C under 4 h reaction. This result indicates that the progressive decomposition of SL-Ni(OH) 2 nanosheets in the formamide occurs during solvothermal reaction, most likely owing to coordination of N groups of formamide molecules with Ni 2+ ions of SL-Ni(OH) 2 nanosheets. Altogether, the reaction time and temperature should be restricted to avoid decomposition of SL-Ni(OH) 2 nanosheets, while the added amount of KOH that determines the reduction rate of Pt precursors has to be controlled to benefit the heterogeneous growth of 1D Pt NWs on the surfaces of SL-Ni(OH) 2 nanosheets. The presence of DS-stabilized SL-Ni(OH) 2 nanosheets appears to be another prerequisite for producing the immobilized Pt NWs. As displayed in Fig. 3a , only spherical Pt NPs with diameters ranging from 1.5 to 3 nm are prepared in the absence of SL-Ni(OH) 2 sheets. Furthermore, both DS-intercalated Ni(OH) 2 nanosheets without fully exfoliation ( Supplementary Fig. 10 ) and carbonate (CO 3 2− )-intercalated Ni(OH) 2 multilayered nanosheets ( Supplementary Fig. 11 ) are prepared as the contrast substrates to compare with SL-Ni(OH) 2 nanosheets. It is evident that as for DS-intercalated Ni(OH) 2 nanosheets without fully exfoliation, Pt NP aggregates are produced and separated from the Ni(OH) 2 nanosheets ( Fig. 3b ); while larger amount of Pt NPs with the diameters of around 5 nm are grown on the surfaces of CO 3 2− -intercalated Ni(OH) 2 multilayered nanosheets ( Supplementary Fig. 12 ). On the basis of the above results from the control experiments, we deduce that SL-Ni(OH) 2 nanosheets affect the formation of Pt NWs through the following aspects: (1) Unique chemical environment of DS-stabilized SL-Ni(OH) 2 nanosheets is indispensible for formation of Pt NWs. The high-resolution N 1 s and S 2p XPS spectra (black curves in Fig. 3c,d ) of SL-Ni(OH) 2 reveal that both formamide (-CONH 2 , 398.8 eV) and DS ions (-SO 3 2− , 167.7 eV) are adsorbed on the SL-Ni(OH) 2 surfaces. Additional N 1 s peak located at 401.5 eV in SL-Ni(OH) 2 corresponds to amide groups of formamide that interact with sulfonic groups in DS ions on the surface of SL-Ni(OH) 2 (ref. 50 ). Meanwhile, this interaction between amide group and sulfonic groups is also recognized in the XPS spectrum of S 2p region, a peak located at 168.9 eV (ref. 50 ). After growth of Pt NWs on the surface of SL-Ni(OH) 2 nanosheets, a new peak appears at 399.2 eV that is attributed to the N-Pt bond (green curve in Fig. 3c ) [24] . While for S element, the peaks with obviously reduced intensity suggest the replacement of the adsorbed DS ions with Pt NWs (green curve in Fig. 3d ). Evidently, the interaction between formamide molecules with DS ions on the surface of SL-Ni(OH) 2 is crucial for generation of ultrathin Pt NWs [27] , [44] . We also notice that similar phenomenon was found in growth of ultrathin gold nanowires on single-layered graphene oxide (GO) nanosheets, in which the absorbed 1-amino-9-octadecene molecules on GO surfaces guided the anisotropic growth of gold nanowires [27] . In our system, as a comparison, CO 3 2− -intercalated Ni(OH) 2 nanosheets in formamide do not exhibit the corresponding peaks at 401.5 or 168.9 eV (red curves in Fig. 3c,d ), suggesting that there is no specific interactions occurring between CO 3 2− and formamide. As a result, the Ni(OH) 2 nanosheets could not be fully exfoliated by using CO 3 2− ions, and only Pt NPs are grown on the surfaces of CO 3 2− -intercalated multilayered Ni(OH) 2 nanosheets ( Supplementary Fig. 12 ). (2) When DS-intercalated Ni(OH) 2 nanosheets are exfoliated to single layers, their surface energy will be greatly enhanced, resulting in much stronger adsorption capability towards Pt precursor ions [24] . The increased adsorption ability guarantees heterogeneous nucleation and growth of Pt on the SL-Ni(OH) 2 nanosheets. (3) Compared with multilayered systems, SL-Ni(OH) 2 nanosheets, which possess higher defect tolerance ability, could allow for horizontal growth of anisotropic nanostructures through slight adjustment of their crystal structure [51] . 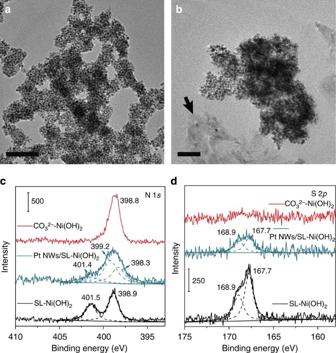Figure 3: TEM and XPS analysis of contrast experiments. (a) TEM image of Pt NPs synthesized without SL-Ni(OH)2; (b) TEM image of Pt NPs/Ni(OH)2synthesized in the presence of DS-intercalated Ni(OH)2without fully exfoliation, and the black arrow points to Ni(OH)2sheets; (c,d) XPS spectra of N 1 s and S 2p region of CO32−-intercalated Ni(OH)2, Pt NWs/SL-Ni(OH)2and SL-Ni(OH)2. Figure 3: TEM and XPS analysis of contrast experiments. ( a ) TEM image of Pt NPs synthesized without SL-Ni(OH) 2 ; ( b ) TEM image of Pt NPs/Ni(OH) 2 synthesized in the presence of DS-intercalated Ni(OH) 2 without fully exfoliation, and the black arrow points to Ni(OH) 2 sheets; ( c , d ) XPS spectra of N 1 s and S 2p region of CO 3 2− -intercalated Ni(OH) 2 , Pt NWs/SL-Ni(OH) 2 and SL-Ni(OH) 2 . Full size image Electrocatalytic performance of Pt NWs/SL-Ni(OH) 2 The HER electrocatalytic activity of as-synthesized Pt NWs/SL-Ni(OH) 2 is evaluated using a rotating disc electrode in 1 M KOH solution at a scan rate of 10 mV s −1 with a rotation rate of 1,600 r.p.m. at room temperature ( Fig. 4a,b ). As comparison, the electrocatalytic activities of other typical nanocatalysts including commercial Pt catalyst (Johnson Matthey, 20 wt.% Pt on activated carbon, referred to Pt/C), Pt NPs/SL-Ni(OH) 2 ( Supplementary Fig. 8 ) and pure ultrathin Pt NWs were also investigated at the same conditions. Pure ultrathin Pt NWs with average diameter of ~2.0 nm ( Supplementary Fig. 13 ) were prepared by using N, N-dimethylmethanamide as both reductant and solvent [44] . Seen from Fig. 4a , it is clear that the HER current density normalized by ECSA of Pt species (for example, −0.07 V versus reversible hydrogen electrode (RHE)) at Pt NWs/SL-Ni(OH) 2 (2.48 mA cm −2 ) is much higher than that at Pt NPs/SL-Ni(OH) 2 (1.06 mA cm −2 ), commercial Pt/C (0.296 mA cm −2 ) and pure Pt NWs (0.381 mA cm −2 ). Interestingly enough, the HER activity of Pt NWs/SL-Ni(OH) 2 is almost one order of magnitude higher than that of the commercial Pt/C catalyst. Even for the Pt/C catalyst modified by electrochemically deposited Ni(OH) 2 (Pt/C@Ni(OH) 2 ), the HER activity (0.692 mA cm −2 at −0.07 V versus RHE) is still far below that of Pt NWs/SL-Ni(OH) 2 ( Supplementary Fig. 14 ). In addition, HER electrocatalytic activity in less alkaline condition (0.1 M KOH) is investigated ( Fig. 4b ), and remarkably the HER current density at Pt NWs/SL-Ni(OH) 2 (6.31 mA cm −2 at −0.07 V versus RHE) is also much higher than that at Pt NPs/SL-Ni(OH) 2 (1.86 mA cm −2 ), commercial Pt/C (0.662 mA cm −2 ) and pure Pt NWs (0.969 mA cm −2 ). The HER current density normalized by the mass of Pt species is further demonstrated in Supplementary Fig. 15 . The mass current density (at −0.07 V versus RHE) of Pt NWs/SL-Ni(OH) 2 is 0.679 mA μg Pt −1 in 1 M KOH and 1.59 mA μg Pt −1 in 0.1 M KOH solution, which is 4.35 and 4.50 times than that of commercial Pt/C, respectively. It is worth mentioning that to our best knowledge, with respect to the important parameters of HER performance (current density at −0.07 V versus RHE and overpotential at 4 mA cm −2 ), the Pt NWs/SL-Ni(OH) 2 hybrids outperform the currently reported electrocatalyst systems ( Supplementary Table 1 ). The reason for the superior HER activity of Pt NWs/SL-Ni(OH) 2 in basic condition should be ascribed to two major factors: (i) combination of Pt with Ni(OH) 2 greatly enhances the HER activity of Pt species (Pt NWs/SL-Ni(OH) 2 versus commercial Pt/C and pure Pt NWs). In the hybrid systems, Ni(OH) 2 substrates can effectively activate the HO-H bond, which remedy the limited capability of Pt in water dissociation in basic solution for HER [8] , [23] . (ii) Ultrathin 1D Pt NWs may expose more active sites while maintaining improved electrons transport characteristics, compared with 0D Pt NPs, Pt NPs/Ni(OH) 2 and Pt/C@Ni(OH) 2 (ref. 38 ). Smaller charge transfer resistance of Pt NWs/SL-Ni(OH) 2 confirmed by electrochemical impedance spectroscopy further demonstrates this improved electron transport property in 1D Pt NWs ( Supplementary Fig. 16 and Supplementary Note 2 ). 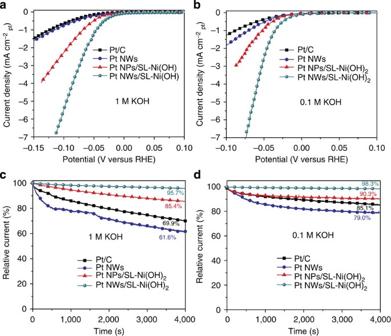Figure 4: Electrocatalytic activity and stability of Pt NWs/SL-Ni(OH)2hybrid materials. (a) HER activity of Pt NWs/SL-Ni(OH)2, Pt NPs/SL-Ni(OH)2, pure Pt NWs and commercial Pt/C (20 wt% Pt) in 1 M KOH at room temperature; (b) HER activity of Pt NWs/SL-Ni(OH)2, Pt NPs/SL-Ni(OH)2, Pt NWs and commercial Pt/C (20 wt.%) in 0.1 M KOH at room temperature. The polarization curves in (a,b) were recorded at a scan rate of 10 mV s−1and a rotation rate of 1,600 r.p.m., and all the current density was normalized by the electrochemical surface areas of Pt. (c) and (d) Normalized current-time (i–t) chronoamperometric responses for HER at Pt NWs/SL-Ni(OH)2, Pt NPs/SL-Ni(OH)2Pt NWs and commercial Pt/C (20 wt.%) electrodes in 1 and 0.1 M KOH solution. Figure 4: Electrocatalytic activity and stability of Pt NWs/SL-Ni(OH) 2 hybrid materials. ( a ) HER activity of Pt NWs/SL-Ni(OH) 2 , Pt NPs/SL-Ni(OH) 2 , pure Pt NWs and commercial Pt/C (20 wt% Pt) in 1 M KOH at room temperature; ( b ) HER activity of Pt NWs/SL-Ni(OH) 2 , Pt NPs/SL-Ni(OH) 2 , Pt NWs and commercial Pt/C (20 wt.%) in 0.1 M KOH at room temperature. The polarization curves in ( a , b ) were recorded at a scan rate of 10 mV s −1 and a rotation rate of 1,600 r.p.m., and all the current density was normalized by the electrochemical surface areas of Pt. ( c ) and ( d ) Normalized current-time (i–t) chronoamperometric responses for HER at Pt NWs/SL-Ni(OH) 2 , Pt NPs/SL-Ni(OH) 2 Pt NWs and commercial Pt/C (20 wt.%) electrodes in 1 and 0.1 M KOH solution. Full size image Finally, the stability of Pt NWs/SL-Ni(OH) 2 , Pt NPs/Ni(OH) 2 , pure Pt NWs and commercial Pt/C during HER process is evaluated by using the steady carbon fibre paper (CP) as a working electrode ( Supplementary Fig. 17 ). Impressively, the chronoamperometric study indicates that, under the same conditions, the current density at as-synthesized Pt NWs/SL-Ni(OH) 2 shows a considerably slower decay than that at Pt/C, pure Pt NWs and Pt NPs/SL-Ni(OH) 2 both in 1 and 0.1 M KOH ( Fig. 4c,d ). Through analysing data shown in Fig. 4c,d , several conclusions can be achieved about the stability performance of Pt NWs/SL-Ni(OH) 2 catalysts. First of all, on the SL-Ni(OH) 2 substrates, the ultrathin 1D Pt NWs have higher stability compared with Pt NPs. Pt NWs/SL-Ni(OH) 2 preserves 95.7 and 98.3% of its initial activity in 1 M and 0.1 M KOH, respectively, after 4,000 s test, while Pt NPs/SL-Ni(OH) 2 keeps 85.4 and 90.3% of the initial activity. The excellent electrochemical stability of 1D nanostructures have been demonstrated by several previous reports [35] , [40] , [52] . It is widely accepted that the asymmetry of 1D ultrathin structure can effectively suppress physical ripening and dissolution during long-term application. Second, the SL-Ni(OH) 2 nanosheets may greatly enhance the HER stability in basic environment. Without the combination of SL-Ni(OH) 2 , pure Pt NWs only maintain 61.6 and 79.0% of its initiate activity in 1 and 0.1 M KOH after 4,000 s test. Third, Pt catalysts in lower concentration of KOH solution possess higher HER stability. Especially for commercial Pt/C and pure Pt NWs, their normalized current remains about 85.1 and 79.0% in 0.1 M KOH after 4,000 s test, which is much >69.9 and 61.6% in 1 M KOH; whereas, for Pt NWs/SL-Ni(OH) 2 and Pt NPs/SL-Ni(OH) 2 , the corresponding variation is much smaller compared with commercial Pt/C and pure Pt NWs. These differences further confirm that the SL-Ni(OH) 2 could effectively improve the HER stability of Pt nanostructures in strong basic environment. Moreover, to investigate the long-term HER stability of Pt NWs/SL-Ni(OH) 2 , we carried out 40,000 s test in both 1 and 0.1 M KOH. As displayed in Supplementary Fig. 18 , Pt NWs/SL-Ni(OH) 2 keeps 82.9 and 92.5% of its initial activity in 1 and 0.1 M KOH after 40,000 s test. These data highlight the superior stability of Pt NWs/SL-Ni(OH) 2 with respect to commercial Pt/C and pure Pt NWs. Supplementary Fig. 18c,d presents typical TEM images of Pt NWs/SL-Ni(OH) 2 after 40,000 s test in 1 M KOH. Generally, the Pt NWs maintain their initial 1D ultrathin nanostructures. There also appear some aggregates and shorter Pt NWs, and this morphology change that gives rise to partial loss of initial active centres should be responsible for decrease of the HER activity after long-time electrolysis. In summary, a facile wet-chemical method is developed to in situ grow ultrathin 1D Pt NWs on single-layered 2D Ni(OH) 2 nanosheets. Benefitting from the unique morphological and structural features including high crystallinity, easy charge transport and strong coupling between the immobilized Pt NWs and the Ni(OH) 2 nanosheets, the Pt NWs/SL-Ni(OH) 2 hybrid materials exhibit the record high electrocatalytic activity for HER in alkaline solution, which is 4–5 times higher than the commercial Pt/C catalyst. Such novel hybrid nanoarchitecture with 1D NWs on single-layered 2D nanosheets not only ensures controllable construction of many artificial materials of varied compositions, geometries and arrangement patterns, but also provides great opportunity for production of the exceptional properties and functionalities [53] , [54] , [55] , [56] , [57] . Chemicals Ni(NO 3 ) 2 ·6H 2 O (99.9%, AR grade) was bought from Sinopharm Chemical Reagent. Urea (99.99%, AR grade) and hexamethylenetetramine (HMT, 99.9%, AR grade) were purchased from Aladdin Reagent. Sodium dodecyl sulfate (SDS, 99.0%, AR grade) and formamide (99.0%, AR grade) were purchased from Xilong Chemical Regent. K 2 PtCl 4 (46-47% Pt, AR grade) and KOH (99.98%, AR grade) were bought from Acros Organics. Ultrapure water (Millipore Milli-Q grade) with a resistivity of 18.2 Mω was used in all the experiments. Synthesis of single-layered Ni(OH) 2 (SL-Ni(OH) 2 ) Preparation of SL-Ni(OH) 2 formamide dispersion was based on the reported method with slight modification [33] . First of all, layered Ni(OH) 2 intercalated with DS was synthesized by precipitation of an aqueous solution of Ni 2+ and SDS through hexamethylenetetramine (HMT) hydrolysis. Three aqueous solutions (0.5 M Ni(NO 3 ) 2 ·6H 2 O, 0.25 M SDS and 1 M HMT solutions) were prepared, and then the Ni 2+ (4 ml), SDS (40 ml) and HMT (12 ml) solutions were mixed in a 200 cm 3 Teflon vessel with Milli-Q water (18 mΩ, 44 ml). The mixed solution was heated at 120 °C for 24 h under airtight condition. After the reaction, the precipitates obtained were centrifuged, washed with water and ethanol, and dried at room temperature ( Supplementary Fig. 10 presented their typical SEM and TEM images). The precipitates (100 mg) were mixed with formamide (50 ml) to exfoliate the host layers, and the resulting suspension was ultrasonicated for 12 h. Subsequently, the suspension was centrifuged (2,000 r.p.m. ), and the supernatants were used as the SL-Ni(OH) 2 formamide dispersion. Detailed characterization was shown in Supplementary Fig. 1 . Synthesis of Carbonate (CO 3 2− )-intercalated Ni(OH) 2 multilayered nanosheets Carbonate (CO 3 2− )-intercalated Ni(OH) 2 multilayered nanosheets were synthesized similar to layered Ni(OH) 2 intercalated with DS without adding SDS. Although CO 3 2− -intercalated Ni(OH) 2 was hardly exfoliated to single layer, its formamide suspension (2 mg ml −1 ) was also treated under ultrasonication for 12 h. Supplementary Fig. 11 presented the typical TEM images of Ni(OH) 2 multilayered nanosheets. Synthesis of Pt NWs/SL-Ni(OH) 2 Three hundred microlitres of K 2 PtCl 4 (60 mM) and 50 μl KOH (5 M) water solution were added to 10 ml SL-Ni(OH) 2 formamide dispersion (0.5 mg ml −1 ), respectively. After that, the mixture was subjected to solvothermal treatment in a 20-ml Teflon-lined autoclave at 120 °C for 4 h to obtain Pt NWs/SL-Ni(OH) 2 products. Synthesis of Pt NPs/SL-Ni(OH) 2 Three hundred microlitres of K 2 PtCl 4 (60 mM) and 5 μl KOH (5 M) water solution were added to 10 ml SL-Ni(OH) 2 formamide dispersion (0.5 mg ml −1 ), respectively. After that, the mixture was subjected to solvothermal treatment in a 20-ml Teflon-lined autoclave at 120 °C for 4 h to obtain Pt NPs/SL-Ni(OH) 2 product. The typical TEM images and XPS analysis of as-synthesized Pt NPs/SL-Ni(OH) 2 were shown in Supplementary Fig. 8 , and the Pt content in Pt NPs/SL-Ni(OH) 2 was quantitatively measured to be about 40.2 wt.% by an ICP-MS technique. Synthesis of Pt NPs/Ni(OH) 2 Three hundred microlitres of of K 2 PtCl 4 (60 mM) and 50 μl KOH (5 M) water solution were added to 10 ml Ni(OH) 2 multilayered nanosheets formamide suspension (0.5 mg ml −1 ), respectively. After that, the mixture was subjected to solvothermal treatment in a 20-ml Teflon-lined autoclave at 120 °C for 4 h to prepare Pt NPs/Ni(OH) 2 . Synthesis of Pure Pt NWs Pure Pt NWs were prepared according to ref. 44 . In brief, 100 mg of H 2 PtCl 6 solution (8 wt. %) and 500 mg of KOH were added to a mixed solution containing 4 ml of ethylene glycol (EG) and 6 ml of N, N-dimethylmethanamide (DMF). After magnetic stirring for 12 h, the resultant homogeneous and transparent solution was transferred into a 25-ml Teflon-lined autoclave. The autoclave was maintained at 170 °C for 8 h and then cooled to room temperature. The black products were collected and washed with ethanol and pure water several times before drying at 80 °C overnight. Typical TEM images of as-synthesized Pt NWs were shown in Supplementary Fig. 13 . Synthesis of Pt/C@Ni(OH) 2 Electrochemically deposited Ni(OH) 2 clusters on Pt/C surfaces were prepared according to ref. 8 . Characterization TEM was performed on a FEI Tecnai G2 F20 electron microscope operated at 200 kV, and the surface morphology was observed under a Hitachi S4800 scanning electron microscope (SEM). Powder XRD patterns were recorded on a Panaltical X’Pert-pro MPD X-ray power diffract meter by using Cu Kα radiation ( λ =1.54056 Å). XPS spectra were performed by an ESCALAB 250 Xi XPS system of Thermo Scientific, where the analysis chamber was 1.5 × 10 −9 mbar and the X-ray spot was 500 μm. AFM measurements were implemented by using a Vecco Dimension 3100 SPM system. Electrochemical measurements The catalyst dispersion or ink was prepared by mixing certain amount of catalysts in 765 μl of water, 200 μl of ethanol and 35 μl of 5 wt % Nafion solution followed by ultrasonication for 1 h. For fabrication of the working electrodes of Pt NWs/SL-Ni(OH) 2 , Pt NPs/SL-Ni(OH) 2 , Pt/C or pure Pt NWs, 5 μl of catalyst ink was loaded onto a glassy carbon electrode of 5 mm in diameter. These electrodes were dried at room temperature. To make our tests more rigorous, actual mass concentrations of the Pt species in catalyst inks were determined by ICP-MS, which were 0.820 mg Pt ml −1 , 0.686 mg Pt ml −1 , 0.856 mg Pt ml −1 and 0.632 mg Pt ml −1 in Pt/C, pure Pt NWs, Pt NPs/SL-Ni(OH) 2 and Pt NWs/SL-Ni(OH) 2 , respectively. Therefore, the actual loading amount of Pt/C, pure Pt NWs, Pt NPs/SL-Ni(OH) 2 and Pt NWs/SL-Ni(OH) 2 was 4.10, 3.43, 4.28 and 3.16 μg, respectively. The accurate measurement of the Pt loading amount was used to determine the ECSA of catalysts and the normalized HER current density by mass of Pt. The electrochemical tests were performed in a three-electrode electrochemical cell (Pine Instruments) using a Pt wire and a Ag/AgCl electrode as a counter and a reference electrode, respectively. Before measurement, a fresh batch of electrolyte with required concentration (0.1 or 1 M) was prepared in a polypropylene bottle by dissolving the required mass of KOH in Milli-Q water. Subsequently, N 2 gas was purged through the solution to achieve an O 2 -free condition. The ECSA was obtained by integrating the H-desorption region of Pt species in 0.1 M KOH and dividing the resulting coulombic charge by 210 C cm Pt −2 (refs 15 , 16 ). All the samples were tested at least for three times to get corresponding average values of ECSA. As shown in Supplementary Fig. 19 , the ECSA value of commercial Pt/C, pure Pt NWs, Pt NPs/SL-Ni(OH) 2 and Pt NWs/SL-Ni(OH) 2 was 52.5±2.2, 40.7±3.5, 27.6±1.5 and 22.8±1.1 m 2 g Pt −1 , respectively. For HER tests, polarization curves were recorded between −0.2 and 0.2 V versus RHE at a scan rate of 10 mV s −1 and a rotation rate of 1,600 r.p.m. at rotating disc electrode. The solution resistances of 0.1 and 1 M KOH measured at room temperature were 44 Ω and 6 Ω, respectively. These resistance values were subsequently used for the IR-correction of the potential recorded in the HER polarization experiments. For stability test, we built an experimental device using CP as a working electrode (shown in Supplementary Fig. 17 ). For our stability tests, CP was cut into 1 × 1 cm 2 plate, and then 25 μl catalyst ink was dropped on it and completely dried at room temperature. The stability of commercial Pt/C, pure Pt NWs, Pt NPs/SL-Ni(OH) 2 and Pt NWs/SL-Ni(OH) 2 during HER process was evaluated by a chronoamperometric method both in 1 M KOH solution (applied potential was −0.077 V versus RHE) and 0.1 M KOH (applied potential was −0.086 V versus RHE). How to cite this article: Yin, H. et al . Ultrathin platinum nanowires grown on single-layered nickel hydroxide with high hydrogen evolution activity. Nat. Commun. 6:6430 doi: 10.1038/ncomms7430 (2015).